The Parkinson’s-associated protein DJ-1 regulates the 20S proteasome The Parkinson’s-associated protein, DJ-1, is a highly conserved homodimer, ubiquitously expressed in cells. Here we demonstrate that DJ-1 is a 20S proteasome regulator. We show that DJ-1 physically binds the 20S proteasome and inhibits its activity, rescuing partially unfolded proteins from degradation. Consequently, DJ-1 stabilizes the cellular levels of 20S proteasome substrates, as we show for α-synuclein and p53. Furthermore, we demonstrate that following oxidative stress, DJ-1 is involved in the Nrf2-dependent oxidative stress response that leads to the upregulation of both the 20S proteasome and its regulator, NQO1. Overall, our results suggest a regulatory circuit in which DJ-1, under conditions of oxidative stress, both upregulates and inhibits the 20S proteasome, providing a rigorous control mechanism at a time when the 20S proteasome becomes the major proteolytic machinery. Such a tight regulation of the 20S proteasome may sustain the balance between the need to rapidly eliminate oxidatively damaged proteins and maintain the abundance of native, intrinsically unstructured proteins, which coordinate regulatory and signalling events. DJ-1 is a small protein of 189 amino acids that is ubiquitously expressed in almost all cells and tissues, including the brain, and exists as a homodimer that is localized to the cytoplasm, mitochondria and nucleus (for reviews, see refs 1 , 2 ). Belonging to the ThiJ/PfpI protein superfamily, DJ-1 is highly conserved, with homologues distributed across all biological kingdoms [3] . DJ-1 was originally identified as an oncogene and its expression was found to be upregulated in several malignancies including breast, lung and prostate cancer. DJ-1 was also implicated in additional disorders such as ischaemic injury, amyotrophic lateral sclerosis [4] , [5] , fertility control and androgen receptor regulation [2] . A decade ago, it was realized that missense, truncation and splice site mutations in DJ-1 all lead to an autosomal recessive, early-onset familial form of Parkinson’s disease (PD; reviewed in refs 2 , 6 ). The specific role of the protein in the pathogenesis of PD is still unclear; however, the diversity of disease states in which DJ-1 is implicated suggests its involvement in a fundamental biological process. Models of DJ-1 deficiency or overexpression have provided evidence that the protein takes part in the oxidative stress response [7] , [8] . It was shown to protect cells from reactive oxygen species, reduce protein misfolding and stabilize mitochondrial potential and morphology. Under oxidative stress, a conserved cysteine residue in DJ-1 (Cys106) is oxidized into cysteine sulfinate and cysteine sulfonate [2] . This oxidative modification is thought to enable DJ-1 to act as a sensor of cellular redox homeostasis, and to participate in cytoprotective signalling pathways in the cell. In addition, oxidative stress was found to induce the rapid relocalization of DJ-1 to mitochondria [7] , [9] , suggesting that mitochondria could be a site for DJ-1’s neuroprotective activity. To date, the molecular function of DJ-1 is still not clear, though a range of biochemical and cellular activities have been proposed for it. These include roles as a cysteine protease [10] , redox-regulated chaperone [11] and transcription modulator [12] , as well as involvement in anti-apoptotic signalling processes [13] , [14] and RNA regulation [15] . DJ-1 was also shown to upregulate glutathione synthesis and heat shock proteins [16] , alter dopamine receptor signalling [17] and coordinate p53 signalling [18] , [19] . Overall, despite the broad interest and impressive progress that has been made in DJ-1 characterization, its key biological functions, and direct and indirect biological implications, remain unclear. Here we combined biochemical and native mass spectrometry approaches, together with cell biology methods, to study the molecular function of DJ-1. Our results revealed that DJ-1 is a regulator of the ubiquitin-independent 20S proteasomal degradation pathway. In general, substrates of the 20S proteasome are composed of proteins containing unstructured or relatively unfolded regions [20] . This class of proteins can be degraded by two alternative proteasomal degradation mechanisms, which are not mutually exclusive: ubiquitin-dependent degradation by the 26S proteasome and ubiquitin-independent degradation by the 20S proteasome. Degradation by the 26S proteasome, which is composed of the 19S and 20S particles, is an active process that is regulated by a series of enzymes that ubiquitinate the substrate and sensitize it to degradation [21] . In contrast, degradation by the 20S proteasome is a passive process that does not require ubiquitin tagging, ATP hydrolysis or the presence of the 19S regulatory particle; rather, it relies on the inherent disorder of the protein being degraded [20] . Many key regulatory proteins such as the tumour suppressors p53 and p73, tau, α-synuclein and the cell cycle regulators p27 and p21 have been shown to be substrates of the 20S proteasome [20] . Moreover, under oxidative conditions, the 20S proteasome was identified as the major degradation machinery [22] , [23] , [24] , [25] . Therefore, it is reasonable to assume that this degradation route would be tightly regulated [26] , [27] , [28] , [29] , as established in the present study. Here we demonstrate that DJ-1 physically binds to the 20S proteasome and inhibits its activity. As a consequence, it can protect various intrinsically unstructured proteins such as p53 and α-synuclein from degradation and stabilize their cellular levels. Our data also indicate that DJ-1’s conserved cysteine residue, Cys106, is essential for this activity, and that protein functionality is preserved, regardless of whether this residue is reduced (Cys-OH) or oxidized to sulfinic acid (Cys-SO 2 − ). In addition, we show that following oxidative stress, DJ-1 is involved in the upregulation of Nrf2, the 20S proteasome regulator NAD(P)H:quinone-oxidoreductase-1 (NQO1) and the 20S proteasome. Combining these findings with those of previous studies uncover a regulatory circuit that highlights the mechanism by which the function of the 20S proteasome is tightly controlled in response to oxidative stress, when proteolysis is highly dependent on this degradation machinery. DJ-1 and NQO1 share structural and functional similarities A clue to the biochemical function of DJ-1 came from examining its three-dimensional structure [30] . We noticed that DJ-1 is similar in structure to NQO1 (ref. 31 ). Both the proteins are active as homodimers and adopt a flavodoxin-like fold consisting of a twisted central parallel β-sheet, sandwiched by α-helical layers ( Supplementary Fig. 1 ) [30] , [31] . Notably, DJ-1 and NQO1 also share a wide spectrum of other features. For example, both DJ-1 and NQO1 are involved in the cellular defense mechanism against oxidative stress [7] , [8] , [32] , [33] . NQO1 is a cytosolic antioxidant enzyme that reduces cellular quinone levels, a process which is crucial for maintaining the cellular redox state [32] , [33] , while DJ-1 is known to be involved in the oxidative stress response [7] , [8] , though its exact role is still not clear. In addition, the expression of DJ-1 and NQO1 is increased in several types of cancer (reviewed in refs 2 , 33 ), and both are associated with neurodegenerative diseases. In particular, mutations in NQO1 lead to an increased risk of developing Alzheimer’s disease [34] , [35] , while mutations in DJ-1 are linked to familial PD (reviewed in refs 1 , 2 ). NQO1 has recently been shown to bind the 20S proteasome [36] and prevent its proteolytic activity, rescuing intrinsically unstructured proteins such as p53, p63 and p73 from 20S degradation [37] . In view of the remarkable similarities between NQO1 and DJ-1, we were motivated to examine whether DJ-1 is also capable of regulating the 20S proteasome activity. DJ-1 inhibits 20S proteasome-mediated degradation To examine whether DJ-1 can protect substrates from 20S proteasome-mediated degradation, we performed a series of degradation assays using a range of substrates. The substrates were selected to represent the repertoire of proteins known to be susceptible to 20S proteolysis, that is, proteins that contain unstructured regions [20] . We therefore used α-synuclein, the carboxyl-terminal (C-terminal) region of p53 (Cp53, residues 292–393) and a mutational variant of NQO1, P187S, which we previously demonstrated to be partially unfolded, and prone to 20S proteasomal degradation [36] . As a negative control, we used calmodulin, which is not degraded by the 20S proteasome unless being oxidized [38] . The time-dependent degradation assays indicated that in all cases tested, the substrates were stable in the absence of the 20S proteasome ( Fig. 1a ). However, following the addition of highly purified 20S proteaseome particles, all substrates were rapidly degraded. The proteolysis turnover rate ( k cat ) was estimated from the degradation curves, to be in the range of 0.03–0.4 min −1 , depending on the substrate identity, assuming that the assay substrate concentrations are much lower than k m . These values are consistent with previously determined turnover rates of both ubiquitin-dependent [39] and -independent [40] 26S proteasome-mediated degradation. The similar k cat values observed for the different degradation routes may support the view that the major component of the rate-limiting step of proteolysis is embedded in the 20S proteasome activity. 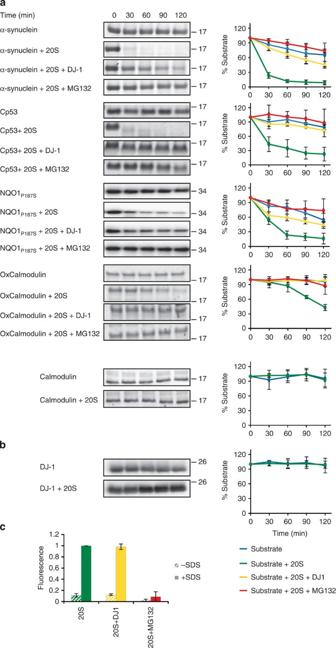Figure 1: DJ-1 inhibits the degradation of partially folded proteins by the 20S proteasome. (a) To examine whether DJ-1 can protect substrates from 20S proteasome proteolysis, we performed a series of time-dependent degradation assays using a range of proteins containing unstructured regions. Intrinsically unstructured proteins such as α-synuclein and the C terminus domain of p53 (Cp53, a.a. 293–393) were used, as well as the mutational variant of NQO1, P187S (NQO1P187S), which we previously demonstrated to be partially unfolded, and prone to 20S proteasomal degradation36. Calmodulin, which becomes a substrate of the 20S proteasome only upon oxidation (OxCalmodulin), served as a control, demonstrating the specificity of the 20S proteasome towards disordered segments. As an additional control, the proteasome inhibitor MG132 was used. At the indicated time points, aliquots were quenched and evaluated by SDS–PAGE (Cp53, α-synuclein and calmodulin) or western blot (NQO1P187S; left panel), followed by quantitative image analysis (right panel). In all tested cases, the substrates were stable in the absence of the 20S proteasome; however, after its addition, they were degraded. In the presence of DJ-1, however, there was a marked decrease in the degradation rate of all substrates. (b) DJ-1 was incubated in the presence and absence of purified 20S proteasomes at the indicated time points, and monitored by western blot analysis, using anti-DJ-1 antibody. The results indicate that unlike the 20S substrates, DJ-1 levels remained constant in the presence of the 20S proteasome. (c) Purified 20S proteasomes were analysed for peptidase activity in the presence and absence of DJ-1 or MG132 using the fluorogenic peptide substrate suc-LLVY-AMC. To enhance the peptidase activity, 0.02% SDS was added to the mixture. Error bars ina–crepresent the s.d. of three repeats. Molecular weights are indicated in the right of each blot in kDa units. Figure 1: DJ-1 inhibits the degradation of partially folded proteins by the 20S proteasome. ( a ) To examine whether DJ-1 can protect substrates from 20S proteasome proteolysis, we performed a series of time-dependent degradation assays using a range of proteins containing unstructured regions. Intrinsically unstructured proteins such as α-synuclein and the C terminus domain of p53 (Cp53, a.a. 293–393) were used, as well as the mutational variant of NQO1, P187S (NQO1 P187S ), which we previously demonstrated to be partially unfolded, and prone to 20S proteasomal degradation [36] . Calmodulin, which becomes a substrate of the 20S proteasome only upon oxidation (OxCalmodulin), served as a control, demonstrating the specificity of the 20S proteasome towards disordered segments. As an additional control, the proteasome inhibitor MG132 was used. At the indicated time points, aliquots were quenched and evaluated by SDS–PAGE (Cp53, α-synuclein and calmodulin) or western blot (NQO1 P187S ; left panel), followed by quantitative image analysis (right panel). In all tested cases, the substrates were stable in the absence of the 20S proteasome; however, after its addition, they were degraded. In the presence of DJ-1, however, there was a marked decrease in the degradation rate of all substrates. ( b ) DJ-1 was incubated in the presence and absence of purified 20S proteasomes at the indicated time points, and monitored by western blot analysis, using anti-DJ-1 antibody. The results indicate that unlike the 20S substrates, DJ-1 levels remained constant in the presence of the 20S proteasome. ( c ) Purified 20S proteasomes were analysed for peptidase activity in the presence and absence of DJ-1 or MG132 using the fluorogenic peptide substrate suc-LLVY-AMC. To enhance the peptidase activity, 0.02% SDS was added to the mixture. Error bars in a – c represent the s.d. of three repeats. Molecular weights are indicated in the right of each blot in kDa units. Full size image Remarkably, in all degradation assays, the presence of DJ-1 led to a vast decrease in the degradation rate of all substrates, reducing the proteasomal k cat value by a factor of nearly 3 for α-synuclein, 2 for both Cp53 and oxidized calmodulin and 1.4 for the mutational variant of NQO1 ( Fig. 1a ). The degradation kinetics curves also indicated that in contrast to the proteasome inhibitor MG132, which completely and uniformly impeded the 20S proteasome, the inhibition efficiency of DJ-1 is dependent on substrate identity. Nevertheless, our results indicate that DJ-1, like NQO1, can indeed rescue a wide variety of partially folded substrates from 20S proteasome degradation. To test whether DJ-1 inhibits protein proteolysis by competing with the substrates, we monitored the stability of DJ-1 following its incubation with the 20S proteasome ( Fig. 1b ). Our analysis shows that the levels of DJ-1 remained the same, regardless of the presence or absence of the 20S proteasome, indicating that it is not degraded by it. We then examined whether the inhibition mechanism of DJ-1 affects the proteasome’s enzymatic capabilities, by performing peptidase activity assays with and without DJ-1 and the proteasome inhibitor MG132 ( Fig. 1c ). While the addition of MG132 almost completely abolished the proteolytic function, no significant change in the peptide degradation capacity of the 20S proteasome was observed in the presence of DJ-1. These observations suggest that unlike MG132, DJ-1 does not block the proteolytic activity of the 20S proteasome; rather it acts by some other molecular mechanism. Whether DJ-1 prevents protein degradation by masking a substrate binding site or by allosteric regulation, remains to be determined. DJ-1 physically binds to the 20S proteasome We next wished to understand whether DJ-1 is capable of preventing degradation by physically interacting with the 20S proteasome, either by binding to the substrate or, alternatively, by forming interactions with both. On the basis of previous observations that point up DJ-1’s chaperone activity [11] , we anticipated that it would bind to 20S proteasome substrates. Accordingly, we applied native mass spectrometry (MS), ion mobility MS (IM-MS) and native gel analysis under a range of experimental conditions, to screen for optimal DJ-1:substrate ratios, incubation times, temperature and buffer solutions. However, we could not detect physical interactions between 20S proteasome substrates and DJ-1, nor any effect on the structural properties of the substrates (the native MS analysis is demonstrated for α-synuclein in Supplementary Fig. 2 ). We then applied the microscale thermophoresis (MST) method, which is based on thermophoresis—the directed motion of molecules in temperature gradients [41] , to measure the intramolecular binding affinity between DJ-1 and the 20S substrate, Cp53. However, no interaction between the two components was observed ( Supplementary Fig. 3a ). Similarly, in a previous study using size-exclusion high-performance liquid chromatography and fluorescence analysis, no evidence for a stable interaction between α-synuclein and DJ-1 was found [42] . Taken together, these findings imply that even if DJ-1 is capable of interacting with 20S substrates, this association is probably transient and unstable, and has no significant effect on substrate conformation. We then analysed the interaction between DJ-1 and the 20S proteasome itself, by means of native MS experiments after mixing the 20S proteasome and DJ-1; free 20S proteasome and DJ-1 were used as controls ( Fig. 2 ). In each of these experiments, the 20S proteasome-associated complexes appeared as a charge state series around 12,000–13,000 m / z , but the peaks were not resolved well enough to unambiguously determine whether DJ-1 was bound to 20S. Therefore, tandem MS (MS/MS) experiments were performed in which a single peak corresponding to ions of the 20S proteasome was isolated. The ions were then subjected to collisional activation, and the individual subunits stripped from the complex were identified. The spectrum recorded for the free 20S proteasome gave rise to the dissociation of α-subunits, consistent with the architecture of this complex, in which the two α 7 ring structures are exposed [21] ( Fig. 2a ). Comparison of this spectrum with that recorded for the 20S proteasome in the presence of DJ-1 revealed additional peaks that correspond in mass to the monomeric form of DJ-1 ( Fig. 2b ). A control MS/MS spectrum of free DJ-1 displayed charge series identical to those that arise when DJ-1 was incubated with the 20S complex ( Fig. 2c ). By extrapolation, we can therefore conclude that before the MS/MS analysis, DJ-1 bound the 20S proteasome. 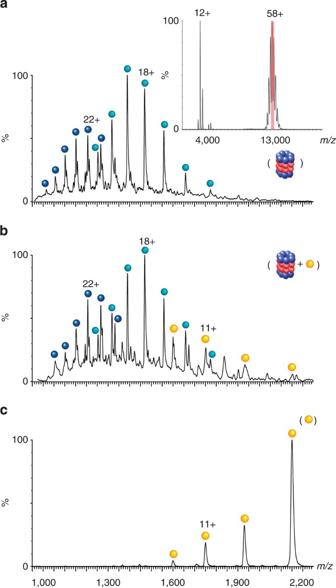Figure 2: DJ-1 physically binds to the 20S proteasome. Free 20S proteasomes (a), 20S proteasomes mixed with DJ-1 (b) and free DJ-1 (c) were examined by native MS. For each sample, the most intense charge state obtained in the MS spectrum was subjected to MS/MS analysis (inset shows the MS spectrum of the free 20S proteasome; the 58+charge state highlighted in red was subjected to MS/MS analysis). Comparison of the free 20S spectrum (a), with that recorded for 20S in the presence of DJ-1 (b), revealed additional peaks that correspond in mass to the monomeric form of DJ-1, as seen in (c). By extrapolation, we can therefore conclude that before MS/MS analysis, DJ-1 binds to the 20S proteasome. Blue and cyan dots correspond to two different α subunits of the 20S proteasome; yellow dots represent monomers of DJ-1. Figure 2: DJ-1 physically binds to the 20S proteasome. Free 20S proteasomes ( a ), 20S proteasomes mixed with DJ-1 ( b ) and free DJ-1 ( c ) were examined by native MS. For each sample, the most intense charge state obtained in the MS spectrum was subjected to MS/MS analysis (inset shows the MS spectrum of the free 20S proteasome; the 58 + charge state highlighted in red was subjected to MS/MS analysis). Comparison of the free 20S spectrum ( a ), with that recorded for 20S in the presence of DJ-1 ( b ), revealed additional peaks that correspond in mass to the monomeric form of DJ-1, as seen in ( c ). By extrapolation, we can therefore conclude that before MS/MS analysis, DJ-1 binds to the 20S proteasome. Blue and cyan dots correspond to two different α subunits of the 20S proteasome; yellow dots represent monomers of DJ-1. Full size image To measure the binding affinity of DJ-1 to the 20S proteasome, we again utilized the MST technology [41] . To this end, we labelled DJ-1 with the NT-647 fluorescent dye, supplemented with increasing concentrations of 20S proteasomes and measured the resulting change in fluorescence. The data indicated that DJ-1 binds the 20S proteasome with an affinity value ( K d ) of 18 nM ( Supplementary Fig. 3b ). Notably, this high-affinity interaction is quite close to the recently determined dissociation constant between the 20S proteasome and the 19S base complex, with a K d value of ~3 nM (ref. 43 ). To further examine the DJ-1/20S proteasome interaction and determine whether DJ-1 is also capable of binding the 26S proteasome, two independent experiments were performed ( Fig. 3 ). Initially, we tested the ability of DJ-1 to interact with purified and functional 26S and 20S proteasomes isolated from rat livers ( Fig. 3a ). Western blot analysis with anti-α4 (a 20S proteasome subunit), anti-RPN2 (a subunit of the 19S particle which, on interaction with the 20S, forms the 26S proteasome) and anti-DJ-1 antibodies revealed that DJ-1 co-migrated with the 20S proteasomes, but not with the 26S proteasomes ( Fig. 3a ). We next validated the existence of this interaction in cells, using a FLAG-tagged β4 subunit of the 20S proteasome, expressed in HEK 293T cells. Cellular extracts were immunoprecipitated (IP) with anti-FLAG, anti-DJ-1 and anti-RPN2 antibodies: the precipitated material was resolved by electrophoresis, and probed with anti-DJ-1, anti-α1 (a 20S proteasome subunit) and anti-RPN2 antibodies. As shown in Fig. 3b , the reciprocal co-IP experiments confirmed the interaction between the 20S proteasome and the endogenous DJ-1. Immunoblot analysis using an antibody directed towards RPN2 gave rise to a faint band when anti-DJ-1 was used for pull down, in comparison with the anti-FLAG co-IP. Likewise, the RPN2 antibody efficiently pulled down the 20S proteasome, but a weak band was observed for DJ-1. These findings may suggest that DJ-1 can bind to 26S proteasomes that are singly capped with the 19S particle (20S–19S), consisting of an exposed 20S proteasome interface. Altogether, these results suggest that DJ-1 has a preference toward binding to the 20S rather than to the 26S proteasome. 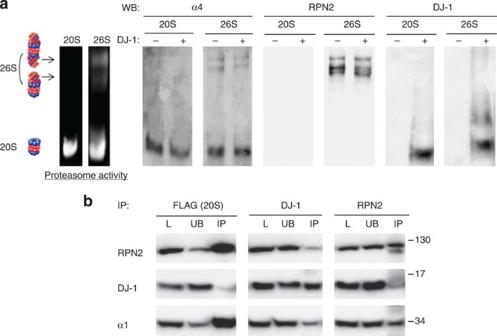Figure 3: DJ-1 preferably binds the 20S proteasome and not the 26S proteasome. (a) 20S and 26S proteasomes purified from rat livers were incubated overnight at 4 °C in the presence (+) or absence (−) of purified recombinant DJ-1. Samples were then separated using 4% native-PAGE, and analysed for peptidase activity, or interaction with DJ-1 by western blot (WB) using anti- α4 (a 20S proteasome subunit), RPN2 (a 19S proteasome subunit) and DJ-1 antibodies. This analysis revealed that DJ-1 co-migrated with the 20S proteasomes, but not with the 26S proteasomes. (b) Lysates of cytosolic proteins from HEK293 cells (L) stably expressing the proteasome β4 subunit tagged with C-terminal FLAG, were subjected to IP using anti-DJ-1 and anti-RPN2 antibodies or anti-FLAG affinity gel and analysed by western blot, using antibodies against DJ-1, α1-subunit and RPN2. Unbound proteins (UB) were run in parallel. The reciprocal co-IP experiments using anti-DJ-1 and anti-FLAG antibodies confirmed the interaction between the 20S complex and DJ-1. The low signal of RPN2 in the DJ-1 IP may indicate that DJ-1 interacts with the singly capped 26S proteasome. Notably, the assay was performed under conditions that preserve the integrity of the 26S proteasome (10% glycerol and 1 mM ATP), as can be seen by the RPN2 bands that appeared when anti-FLAG was used for co-IP. All experiments were repeated at least three times. Figure 3: DJ-1 preferably binds the 20S proteasome and not the 26S proteasome. ( a ) 20S and 26S proteasomes purified from rat livers were incubated overnight at 4 °C in the presence (+) or absence (−) of purified recombinant DJ-1. Samples were then separated using 4% native-PAGE, and analysed for peptidase activity, or interaction with DJ-1 by western blot (WB) using anti- α4 (a 20S proteasome subunit), RPN2 (a 19S proteasome subunit) and DJ-1 antibodies. This analysis revealed that DJ-1 co-migrated with the 20S proteasomes, but not with the 26S proteasomes. ( b ) Lysates of cytosolic proteins from HEK293 cells (L) stably expressing the proteasome β4 subunit tagged with C-terminal FLAG, were subjected to IP using anti-DJ-1 and anti-RPN2 antibodies or anti-FLAG affinity gel and analysed by western blot, using antibodies against DJ-1, α1-subunit and RPN2. Unbound proteins (UB) were run in parallel. The reciprocal co-IP experiments using anti-DJ-1 and anti-FLAG antibodies confirmed the interaction between the 20S complex and DJ-1. The low signal of RPN2 in the DJ-1 IP may indicate that DJ-1 interacts with the singly capped 26S proteasome. Notably, the assay was performed under conditions that preserve the integrity of the 26S proteasome (10% glycerol and 1 mM ATP), as can be seen by the RPN2 bands that appeared when anti-FLAG was used for co-IP. All experiments were repeated at least three times. Full size image DJ-1 C106A does not prevent substrate proteolysis The conserved cysteine residue, Cys106, in DJ-1 is known to be both functionally essential and sensitive to oxidative modification [2] . We therefore wished to investigate whether this residue is also crucial for the ability of DJ-1 to prevent 20S proteasomal degradation. To this end, degradation assays were performed using the 20S proteasome and α-synuclein and Cp53 as substrates, and either WT DJ-1 (DJ-1 WT ) or its mutational variant C106A (DJ-1 C106A ). In the absence of the 20S proteasome, both substrates were stable; however, they were entirely degraded in its presence ( Fig. 4 ). Interestingly, in comparison with DJ-1, which can significantly prevent substrate degradation, the capacity of DJ-1 C106A to inhibit 20S proteolysis was lower by a factor of ~3 ( Fig. 4 ). 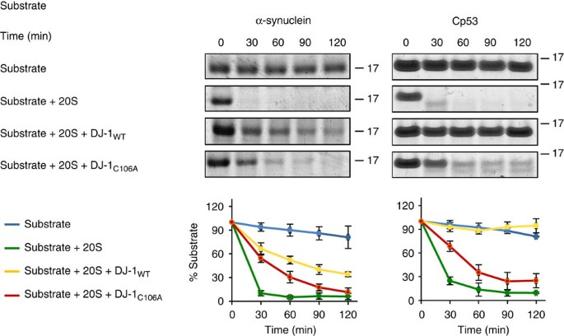Figure 4: DJ-1C106Ais incapable of protecting substrates from 20S proteasomal degradation. Time-dependent 20S proteasome degradation assays of α-synuclein and the C-terminal region of p53 (Cp53, residues 292–393), in the presence or absence of DJ-1WTor DJ-1C106A. At the indicated time points, aliquots were quenched and evaluated by SDS–PAGE (top panel), followed by chemiluminescence quantification (bottom panel). In contrast to DJ-1WT, DJ-1C106Ahas a notably reduced capacity to rescue α-synuclein and Cp53 from degradation. Error bars represent the s.d. of three repeats. Figure 4: DJ-1 C106A is incapable of protecting substrates from 20S proteasomal degradation. Time-dependent 20S proteasome degradation assays of α-synuclein and the C-terminal region of p53 (Cp53, residues 292–393), in the presence or absence of DJ-1 WT or DJ-1 C106A . At the indicated time points, aliquots were quenched and evaluated by SDS–PAGE (top panel), followed by chemiluminescence quantification (bottom panel). In contrast to DJ-1 WT , DJ-1 C106A has a notably reduced capacity to rescue α-synuclein and Cp53 from degradation. Error bars represent the s.d. of three repeats. Full size image We then tested whether the inability of DJ-1 C106A to inhibit proteolysis is due to large conformational changes or partial unfolding of this protein. However, examination of the MS and IM-MS spectra of DJ-1 C106A indicated that they were identical to that obtained for DJ-1 WT (MS spectra are shown in Supplementary Fig. 4 ). We therefore continued by examining the interaction of DJ-1 C106A with the 20S proteasome. MST experiments indicated that DJ-1 C106A interacts with the 20S proteasome with a K d value of 13 nM ( Supplementary Fig. 3c ), very similar to the measured affinity between DJ-1 WT and the 20S particle ( Supplementary Fig. 3b ). Next, a series of tandem MS experiments were conducted after mixing the 20S proteasome with DJ-1 C106A . The acquired MS/MS spectrum of the DJ-1 C106A /20S proteasome ( Supplementary Fig. 5 ) indicated that DJ-1 C106A binds the 20S proteasome; however, the charge state distribution of DJ-1 C106A was significantly broader than that of the wild-type protein ( Fig. 2 ). It was previously demonstrated that the number of charges an ejected monomer accommodates during the dissociation process is correlated with the extent of its unfolding [44] . The key determinants that promote the unfolding of the dissociated monomer are high subunit flexibility, an increased number of interfacial salt bridges and larger interfaces. Hence, the different MS/MS patterns of DJ-1 C106A and the wild-type protein may suggest that they associate with the 20S proteasome in a somewhat different manner. In summary, our findings suggest that although the DJ-1 C106A mutant interacts with the 20S proteasome, it is incapable of inhibiting its activity. Thus, binding to the 20S proteasome per se is not sufficient for inhibiting substrate degradation. DJ-1 inhibits degradation independently of Cys106 oxidation To determine whether the loss of protective function of DJ-1 C106A is due to the absence of Cys106 oxidation or the absence of the cysteine residue itself, we monitored the protein’s ability to inhibit 20S proteasome degradation following oxidative modification. We oxidized DJ-1 using elevated levels of hydrogen peroxide. Following removal of the oxidizing agent, we monitored the ability of DJ-1 to rescue substrates from proteolysis by performing degradation assays using SDS–polyacrlyamide gel (SDS–PAGE) analysis ( Fig. 5a,b and Supplementary Fig. 6 ). In parallel, the oxidation state of DJ-1 WT and DJ-1 C106A was monitored by MS measurements ( Fig. 5c ). 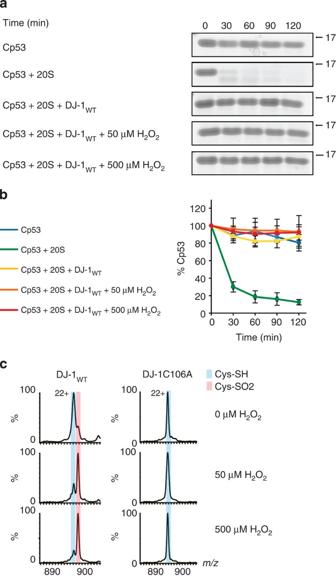Figure 5: Oxidative modification of Cys106 does not abolish the ability of DJ-1 to inhibit the 20S proteasome. (a)In vitro20S proteasome degradation assays of Cp53 in the presence or absence of DJ-1 treated with increasing H2O2concentrations. The oxidative conditions do not affect DJ-1’s ability to rescue Cp53 from 20S proteasome-mediated degradation. Cp53 levels were monitored by Coomassie Blue staining, followed by quantitative image analysis (b). (c) MS analysis of WT DJ-1 and the C106A mutant treated with 0, 50 and 500 μM of H2O2. To emphasize the shifts in mass associated with cysteine thiol (shown by a blue strip) oxidation to sulfinic acid (red strip), only the 22+charge state is shown. The C106A substitution prevents the formation of oxidized DJ-1 isoforms, suggesting that C106 is the residue that is oxidized, whereas the additional DJ-1 cysteines (C46 and C53) remain in their reduced state under the same conditions, consistent with previous published data2. Error bars inbrepresent the s.d. of three repeats. Figure 5: Oxidative modification of Cys106 does not abolish the ability of DJ-1 to inhibit the 20S proteasome. ( a ) In vitro 20S proteasome degradation assays of Cp53 in the presence or absence of DJ-1 treated with increasing H 2 O 2 concentrations. The oxidative conditions do not affect DJ-1’s ability to rescue Cp53 from 20S proteasome-mediated degradation. Cp53 levels were monitored by Coomassie Blue staining, followed by quantitative image analysis ( b ). ( c ) MS analysis of WT DJ-1 and the C106A mutant treated with 0, 50 and 500 μM of H 2 O 2 . To emphasize the shifts in mass associated with cysteine thiol (shown by a blue strip) oxidation to sulfinic acid (red strip), only the 22 + charge state is shown. The C106A substitution prevents the formation of oxidized DJ-1 isoforms, suggesting that C106 is the residue that is oxidized, whereas the additional DJ-1 cysteines (C46 and C53) remain in their reduced state under the same conditions, consistent with previous published data [2] . Error bars in b represent the s.d. of three repeats. Full size image Treating DJ-1 with 50 μM hydrogen peroxide resulted in a mixture of DJ-1 forms ( Fig. 5c ). A minor population of native DJ-1 and a major population of DJ-1 with a 32-Da mass shift was seen, corresponding to the addition of two oxygen atoms, as would be expected from oxidation of cysteine to sulfinic acid (Cys-SO 2 − ). This mass shift was not observed in the DJ-1 C106A mutant, suggesting that Cys106 is indeed the cysteine that undergoes oxidation. This observation is supported by previous findings, which indicated that of the three cysteine residues in human DJ-1 (Cys46, Cys53 and Cys106), Cys106 is the most prone to oxidative modification [2] . Further oxidation of DJ-1 with 500 μM hydrogen peroxide led to an increase in the relative abundance of the sulfinic acid state, in comparison with the non-oxidized protein. Again, no change in mass was detected in the DJ-1 C106A mutant. Nevertheless, regardless of the Cys106 oxidation state, DJ-1 inhibited substrate degradation ( Fig. 5a,b and Supplementary Fig. 6 ). Taken together, these findings indicate that while Cys106 is crucial for DJ-1 inhibitory activity, its reduced or –SO 2 − state does not influence the protein’s activity. DJ-1 stabilizes the cellular levels of 20S proteasome substrates We were motivated to examine whether our in vitro observations, revealing the ability of DJ-1 to inhibit the 20S proteasome, were also relevant within the context of the cellular environment. Therefore, we silenced DJ-1 in HeLa cells and tested the effect on the levels of α-synuclein, a 20S proteasome substrate ( Fig. 6a ). Western blot analysis indicated a reduction in the levels of α-synuclein, which were correlated with the decrease in DJ-1 levels. 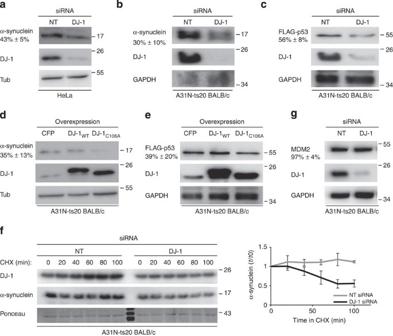Figure 6: DJ-1 stabilizes the cellular levels of 20S proteasome substrates. HeLa and A31N-ts20 BALB/C cells were transiently transfected to silence (a–c) or overexpress DJ-1WTand its mutational variant DJ-1C106A(d,e), with (c,e) or without (a,b,d) FLAG-p53. Forty-eight hours after transfection, A31N-ts20 BALB/C cells were moved to 39 °C. The levels of the different proteins were examined by western blot analyses 72 h post transfection. As controls, non-targeting siRNA (NT) (a–c) or the fluorescent protein Cerulean (CFP) (d,e) were used. The results indicate that silencing DJ-1 or overexpressing the dominant negative DJ-1C106A, reduce the cellular levels of 20S proteasome substrates p53 and α-synuclein. (f) To evaluate the degradation rate of α-synuclein in cells, depleted of DJ-1, a CHX chase was performed, using A31N-ts20 BALB/c cells transfected with siRNA against DJ-1 or non-targeting siRNA. Forty-eight hours after transfection, the cells were moved to 39 °C and 72 h post transfection, CHX was added. Cell extracts were prepared at the indicated times following the drug addition, analysed by immunoblotting and quantified by image analysis. Error bars represent s.e. (g) The impact of DJ-1 knockdown on the stability of MDM2, which is degraded in an ubiquitin-dependent manner by the 26S proteasome, was examined in A31N-ts20 BALB/C cells. After transfection, the cells were grown at 32 °C. Western blot analyses were performed 72 h post transfection with DJ-1 siRNA or non-targeting siRNA (NT). GAPDH, tubulin (Tub) and Ponceau S-staining served as loading controls. The average level of DJ-1 in silenced HeLa and A31N-ts20 cells, relative to its level in non-silenced cells was 22%±4% (n=5) and 23%±4% (n=21), respectively. Percent expression±s.e. of the different proteins, in DJ-1-silenced cells (a–c,g) or in cells overexpressing the mutational variant DJ-1C106A(d,e), relative to control cells was calculated. Values are shown under the name of the proteins tested (α-synuclein ina,b,d, FLAG-p53 inc,eand MDM2 ing) of relevant blots. All experiments were repeated between three and seven times. Figure 6: DJ-1 stabilizes the cellular levels of 20S proteasome substrates. HeLa and A31N-ts20 BALB/C cells were transiently transfected to silence ( a – c ) or overexpress DJ-1 WT and its mutational variant DJ-1 C106A ( d , e ), with ( c , e ) or without ( a , b , d ) FLAG-p53. Forty-eight hours after transfection, A31N-ts20 BALB/C cells were moved to 39 °C. The levels of the different proteins were examined by western blot analyses 72 h post transfection. As controls, non-targeting siRNA (NT) ( a – c ) or the fluorescent protein Cerulean (CFP) ( d , e ) were used. The results indicate that silencing DJ-1 or overexpressing the dominant negative DJ-1 C106A , reduce the cellular levels of 20S proteasome substrates p53 and α-synuclein. ( f ) To evaluate the degradation rate of α-synuclein in cells, depleted of DJ-1, a CHX chase was performed, using A31N-ts20 BALB/c cells transfected with siRNA against DJ-1 or non-targeting siRNA. Forty-eight hours after transfection, the cells were moved to 39 °C and 72 h post transfection, CHX was added. Cell extracts were prepared at the indicated times following the drug addition, analysed by immunoblotting and quantified by image analysis. Error bars represent s.e. ( g ) The impact of DJ-1 knockdown on the stability of MDM2, which is degraded in an ubiquitin-dependent manner by the 26S proteasome, was examined in A31N-ts20 BALB/C cells. After transfection, the cells were grown at 32 °C. Western blot analyses were performed 72 h post transfection with DJ-1 siRNA or non-targeting siRNA (NT). GAPDH, tubulin (Tub) and Ponceau S-staining served as loading controls. The average level of DJ-1 in silenced HeLa and A31N-ts20 cells, relative to its level in non-silenced cells was 22%±4% ( n =5) and 23%±4% ( n =21), respectively. Percent expression±s.e. of the different proteins, in DJ-1-silenced cells ( a – c , g ) or in cells overexpressing the mutational variant DJ-1 C106A ( d , e ), relative to control cells was calculated. Values are shown under the name of the proteins tested (α-synuclein in a , b , d , FLAG-p53 in c , e and MDM2 in g ) of relevant blots. All experiments were repeated between three and seven times. Full size image Taking into account that partly unfolded substrates can be sent to degradation via both the 20S and 26S proteasomes [20] , it was necessary to clarify that the function of DJ-1 is specifically associated with the 20S and not the 26S proteasome degradation route. We therefore silenced the endogenous DJ-1 in the A31N-ts20 BALB/c cell line that harbours a temperature-sensitive E1 variant and, as a consequence, is defective in ubiquitination at the restrictive temperature ( Supplementary Figs 7 and 8 ) [45] . Western blot analyses were performed to detect the levels of the 20S substrates α-synuclein and FLAG-p53, using total protein extracts purified 24 h after transition to the restrictive temperature. Silencing of DJ-1 in these cells resulted in a marked reduction in α-synuclein and FLAG-p53 levels ( Fig. 6b,c ). Similarly, we transfected these cells with plasmids expressing either DJ-1 WT or the DJ-1 C106A mutant ( Fig. 6d,e ). We found that 20S substrate levels were not altered in cells expressing DJ-1 WT , but a clear decrease in their levels was detected in cells expressing DJ-1 C106A . These results indicate that interfering with the normal function of DJ-1 in cells, either by decreasing its levels or by overexpressing a mutant form, thus creating a dominant negative effect, results in reduction in the steady state levels of α-synuclein and p53. Next we sought to evaluate the effect of DJ-1 on the degradation rate of a 20S substrate. We therefore treated A31N-ts20 cells transfected with short interfering RNA (siRNA) targeting DJ-1, with the protein synthesis inhibitor cycloheximide (CHX), and monitored, over time, the decay in the level of α-synuclein, under growth conditions that inhibit ubiquitination ( Fig. 6f ). In addition to the increase in DJ-1 levels, which is consistent with previous observations [46] , [47] , we observed that the α-synuclein pool remained stable when treated with the non-targeting siRNA. However, the knockdown of DJ-1 led to a gradual depletion of the protein on chasing with CHX, further emphasizing the correlation between DJ-1 levels and α-synuclein stability. To determine whether DJ-1 influences the stability of an ubiquitinated substrate, we examined the consequences of DJ-1 downregulation on the levels of the E3 ubiquitin ligase MDM2, which mediates its own ubiquitination and proteasomal targeting [48] . As seen in Fig. 6g , siRNA-mediated depletion of DJ-1 did not affect the cellular levels of MDM2. Taken together, our results support the view that DJ-1 affects the cellular stability of 20S proteasome substrates. DJ-1 activates the 20S proteasome via Nrf2 and NQO1 Previously it was shown that DJ-1 is involved in mediating the activation of Nrf2, the stress-responsive transcription factor [49] . In addition, independent studies have indicated that Nrf2 activation leads to the upregulation of NQO1 (refs 50 , 51 ) and to increased expression of 20S proteasome subunits [30] , [52] , [53] . To determine whether these events are linked, we monitored the levels of Nrf2, NQO1 and the 20S proteasome in control and DJ-1-silenced A31N-ts20 cells treated with diethylmaleate (DEM), a glutathione-depleting compound that causes accumulation of reactive oxygen species within the cell [54] ( Fig. 7 ). We found that in control cells, oxidative stress led to the accumulation of Nrf2 in the nucleus, along with an increase in the levels of cytosolic 20S proteasome and NQO1. In DJ-1-silenced cells, however, the levels of Nrf2 and the 20S proteasome remained steady and the induction of NQO1 was less pronounced. This finding demonstrates that following oxidative stress DJ-1 is involved in the upregulation of Nrf2, NQO1 and 20S proteasome. 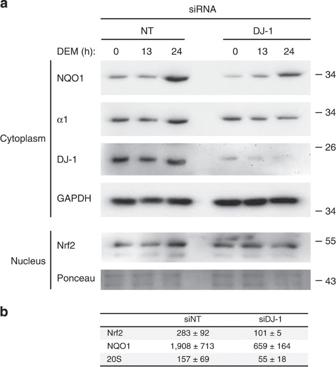Figure 7: DJ-1 is involved in the upregulation of Nrf2, NQO1 and the 20S proteasome activity. (a) A31N-ts20 BALB/C cells grown at 32 °C were transiently transfected with siRNA against DJ-1 or a non-targeting siRNA (NT). Forty-eight hours after transfection, cells were treated with 100 μM DEM and collected at different time points. Cytosolic and nuclear fractions were analysed by western blots to monitor the levels of cytosolic NQO1, α1 (a 20S proteasome subunit), DJ-1 and the nuclear level of Nrf2. GAPDH and Ponceau-S staining served as loading controls. The experiment was repeated three times. (b) The increase in protein levels 24 h after induction of oxidative stress was quantified in respect to T0. Values are an average of three independent experiments, errors represent s.e.. Figure 7: DJ-1 is involved in the upregulation of Nrf2, NQO1 and the 20S proteasome activity. ( a ) A31N-ts20 BALB/C cells grown at 32 °C were transiently transfected with siRNA against DJ-1 or a non-targeting siRNA (NT). Forty-eight hours after transfection, cells were treated with 100 μM DEM and collected at different time points. Cytosolic and nuclear fractions were analysed by western blots to monitor the levels of cytosolic NQO1, α1 (a 20S proteasome subunit), DJ-1 and the nuclear level of Nrf2. GAPDH and Ponceau-S staining served as loading controls. The experiment was repeated three times. ( b ) The increase in protein levels 24 h after induction of oxidative stress was quantified in respect to T0. Values are an average of three independent experiments, errors represent s.e.. Full size image Here we show that DJ-1 rescues partially unfolded proteins from 20S proteasomal degradation, and that its cellular levels influence the stability of 20S proteasome substrates. We also establish that DJ-1 acts by physically associating with the 20S proteasome. This interaction, however, does not perturb the enzymatic activity of the complex. In addition, we demonstrate that the extent of DJ-1 mediated protection from degradation is substrate dependent. The mechanism underlying DJ-1’s ability to inhibit the 20S proteasome remains unclear, though it may resemble that of the 20S proteasome regulator PA200. Like DJ-1, PA200 does not eliminate the peptidase activity of the 20S proteasome; rather, it reduces the ability of the complex to degrade oxidatively damaged proteins [55] , [56] . Considering that an allosteric pathway of communication exists within the 20S proteasome, extending from the α-rings, where the 19S particle binds, to the active sites of the β-rings [57] , [58] , it is tempting to speculate that DJ-1 and perhaps also PA200 function as allosteric regulators. In such a scenario, its interaction with the 20S proteasome would perturb the allosteric path of propagated structural changes, shifting the complex into a proteolytically repressed conformational state. DJ-1 is known to be responsive to oxidative stress, and it is assumed that direct oxidization by free radicals enables it to act as a sensor of cellular redox homeostasis [7] , [8] . In particular, the oxidation of the highly reactive and conserved Cys106 was shown to modulate DJ-1 activity [2] . Our data indicate that both the reduced thiol state (Cys106-OH) and oxidative sulfinate (Cys106-SO 2 − ) forms of Cys106 are functional. These observations are consistent with X-ray crystallography results, demonstrating that DJ-1 structures of the reduced and oxidative sulfinate states are virtually identical [7] , [30] . Thus, it is possible that the sensitivity of Cys106 to oxidative conditions is required for the other known attributes of DJ-1 such as relocalization to mitochondria [7] , [9] or stabilization of Nrf2 (ref. 49 ). Unlike Cys106 oxidation, substituting the Cys106 residue with alanine, however, had a negative impact on DJ-1 activity. Our results demonstrate that even though the mutational variant, DJ-1 C106A , was able to bind the 20S proteasome, it was incapable of preventing 20S proteasomal degradation. The difference in the MS/MS dissociation routes of DJ-1 WT and DJ-1 C106A from the 20S proteasome suggests that they bind the 20S proteasome in rather different ways. However, the structural differences between the two DJ-1 WT or DJ-1 C106A 20S proteasome complexes, and the reasons why Cys106 oxidation maintains the proper binding conformation but its replacement with alanine does not, remain unclear. Like DJ-1, NQO1 is a homodimeric flavodoxin-like protein involved in the defense mechanism against oxidative stress. It acts as a cytosolic oxidoreductase enzyme that reduces quinones and aromatic nitro compounds [32] , [33] . In addition, as demonstrated here for DJ-1, NQO1 binds the 20S proteasome, and rescues proteins containing unstructured domains from 20S proteasomal degradation [36] , [37] . However, unlike DJ-1 that is ubiquitously expressed in various human tissues and is localized in the nucleus, cytoplasm and mitochondria [2] , cytosolic NQO1 expression is induced in response to various stimuli, including antioxidants, xenobiotics and heavy metals [32] , [33] . The antioxidant response element (ARE) in the NQO1 gene promoter is required for its expression and induction [59] . Interestingly, DJ-1 is involved in stimulating the expression of NQO1 (refs 49 , 50 ). The mechanism by which DJ-1 activates NQO1 implicates the stabilization of Nrf2, an oxidative transcription regulator [49] , [50] and a strong activator of ARE-mediated gene expression [59] , [60] . Under normal cellular conditions, Nrf2 is maintained at basal levels in cells by binding to its inhibitor protein, Keap1, which targets Nrf2 for ubiquitination and constitutive degradation by the 26S proteasome [61] . On exposure to oxidative stress, two parallel pathways were shown to stabilize Nrf2. The first involves the inactivation of the 26S proteasome by inducing the dissociation of the complex into its 20S and 19S components [62] , [63] . The second mechanism is mediated by DJ-1, which was shown to stabilize Nrf2 by preventing its association with Keap1 (ref. 49 ). Following its stabilization, Nrf2 translocates to the nucleus [64] , where it forms heterodimers with other transcription regulators such as small Maf proteins, and induces the expression of detoxification enzymes such as NQO1 (refs 59 , 60 ). Without intact DJ-1, the Nrf2 protein is unstable, and transcriptional responses are thereby decreased both basally, and after induction [49] , [50] . Thus, while DJ-1 is capable of directly inhibiting 20S proteasome activity, following oxidative stress, it recruits NQO1 to assist in 20S proteasome regulation. Previous studies have indicated that Nrf2 signalling also takes a role in upregulating the expression of 20S proteasomes [25] , [65] . As demonstrated for NQO1, Nrf2 responds to oxidative stress by binding to ARE or electrophile response elements in the 5′’-untranslated regions of 20S proteasome subunits and induces their expression [25] . These findings, combined with ours ( Fig. 7 ), make it clear that a regulatory circuit tightly controlling the activity of the 20S proteasome is at work ( Fig. 8 ). Within this loop, DJ-1 acts as a bifunctional protein, promoting not only the inhibition of the 20S proteasome, but also its activation. DJ-1 prevents 20S proteasomal degradation by physically binding to the 20S proteasome, as well as by inducing the expression of NQO1 through Nrf2 stabilization. In parallel, an Nrf2 mediated expression of 20S proteasomes occurs. 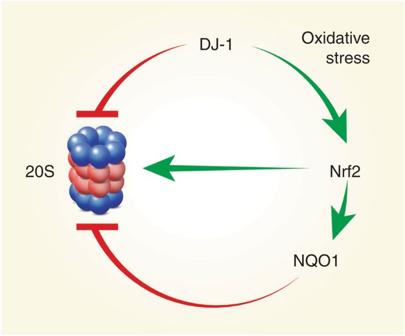Figure 8: DJ-1 regulates 20S proteasome activity. Our results indicate that DJ-1 physically binds the 20S proteasome and inhibits its function, independent of the oxidative modifications of Cys106 to sulfinic acid. Previous studies and our results indicate that under oxidative stress, DJ-1 stabilizes Nrf2, the antioxidant stress response transcription factor, which leads to the expression of NQO1 (refs49,70). NQO1 reinforces the function of DJ-1 by binding to the 20S proteasome and preventing proteolysis36,37. Nrf2, on the other hand, also promotes the expression of 20S proteasome subunits25,65, in accordance with the cell’s need to rapidly eliminate oxidatively damaged proteins. This robust regulatory mechanism is probably necessary to sustain the balance between the need to efficiently eliminate oxidatively damaged proteins, ensure proper proteasomal function and maintain the abundance of the naturally unfolded proteins. Green arrows indicate activation and red lines ending in a bar represent inhibition. Figure 8: DJ-1 regulates 20S proteasome activity. Our results indicate that DJ-1 physically binds the 20S proteasome and inhibits its function, independent of the oxidative modifications of Cys106 to sulfinic acid. Previous studies and our results indicate that under oxidative stress, DJ-1 stabilizes Nrf2, the antioxidant stress response transcription factor, which leads to the expression of NQO1 (refs 49 , 70 ). NQO1 reinforces the function of DJ-1 by binding to the 20S proteasome and preventing proteolysis [36] , [37] . Nrf2, on the other hand, also promotes the expression of 20S proteasome subunits [25] , [65] , in accordance with the cell’s need to rapidly eliminate oxidatively damaged proteins. This robust regulatory mechanism is probably necessary to sustain the balance between the need to efficiently eliminate oxidatively damaged proteins, ensure proper proteasomal function and maintain the abundance of the naturally unfolded proteins. Green arrows indicate activation and red lines ending in a bar represent inhibition. Full size image A logical question that arises is why DJ-1 function seems to entail two opposing feedback mechanisms, upregulation and downregulation of the 20S proteasome activity. The answer probably lies in the critical need to maintain proper 20S proteasomal activity, following oxidative stress. Under these conditions, it is necessary to rapidly degrade oxidized proteins before they can aggregate and threaten cell viability. The 20S proteasome then becomes the major degradation machinery [22] , [27] , [66] , probably due to its higher resistance to oxidation [52] , [53] and the sensitivity of the ubiquitinylation pathway to redox conditions [67] . Yet there remains a need to regulate its activity, as the 20S proteasome can unselectively degrade any protein that contains an unstructured region [20] , including the many intrinsically unstructured proteins involved in signalling and regulation of cellular processes [68] . Among them are the tumour suppressors p53 and p73, tau, α-synuclein and the cell cycle regulators p21 and p27, all of which were shown to be natural substrates of the 20S proteasome [20] . As a consequence, a robust regulatory mechanism is necessary to sustain the balance between the cellular need to rapidly eliminate oxidatively damaged proteins and maintain the abundance of the intrinsically disordered proteins. We suggest that DJ-1 plays an important role in this critical system. Plasmids and proteins The pET-15b-hDJ-1 vector, obtained from Gregory Petsko (Brandeis University), was used as a template for introducing the C106A mutation by Restriction Free Cloning, using the primer pair: forward: 5′-CTGATAGCCGCCATCGCAGCAGGTCCTACTGCTCTG-3′, reverse: 5′-CAGAGCAGTAGGACCTGCTGCGATGGCGGCTATCAG-3′. The presence of the mutation was verified by sequencing. Human DJ-1 fused to a C-terminal HA tag, human DJ-1 C106A , and the Cerulean fluorescent protein (Cer), were cloned into the mammalian expression plasmid pDsRed-monomer-Hyg (Clontech), replacing the DsRed gene. The pCMV-FLAG-p53 plasmid was obtained from Yosef Shaul (Weizmann Institute of Science). A construct containing the C-terminal region of p53 (Cp53, a.a. 293–393) was obtained from Assaf Friedler (Hebrew University of Jerusalem) and purified as described previously [69] . Purified α-synuclein was given to us by Lashuel Hilal (Federal Institutes of Technology). Antibodies For western blot assays, we used rabbit monoclonal anti-DJ-1 (ab76008, Abcam, diluted to 1:3,000), rabbit monoclonal anti-RPN2 (ab2941, Abcam, diluted to 1:1,000), monoclonal anti-FLAG M2 (Sigma F3165, diluted to 1:1,000), mouse monoclonal anti-tubulin (ab7291, Abcam, diluted to 1:5,000), rabbit monoclonal anti-α-synuclein (ab51252, Abcam, diluted to 1:1,000), rabbit monoclonal anti-α4 proteasome subunit, (kindly provided by Chaim Kahana, Weizmann Institute, diluted to 1:10,000), rabbit polyclonal anti-α1 proteasome subunit (ab3325, Abcam, diluted to 1:10,000) and mouse monoclonal anti-GAPDH (47339, Novus, diluted to 1:1,000). For IP experiments, we used goat polyclonal anti-DJ-1 (ab4150, Abcam) and mouse monoclonal anti-FLAG (M2) gel (Sigma-Aldrich). Purification of the 20S proteasome Rat livers were chosen as our source for 20S proteasomes, given the high evolutionary conservation of subunit sequences that exist between human and rat (>96% identity). Purification of the rat 20S proteasome was performed as described previously [36] . In brief, rat livers were homogenized in buffer containing 20 mM Tris-HCL (pH 7.5), 1 mM EDTA, 1 mM dithiothreitol (DTT) and 250 mM sucrose. The extract was subjected to centrifugation, first at 1,000 g for 15 min. The supernatant was then diluted to 400 ml to a final concentration of 0.5 M NaCl and 1 mM DTT and subjected to ultracentrifugation for 2.2 h at 145,000 g . The supernatant was centrifuged again at 150,000 g for 6 h. The pellet containing the proteasomes was resuspended in 20 mM Tris-HCl (pH 7.5) and loaded onto 1.8 L Sepharose 4B resin. Fractions containing the 20S proteasome were identified by their ability to hydrolyse the flurogenic peptide suc-LLVY-AMC, in the presence of 0.02% SDS. Proteasome-containing fractions were then combined and loaded onto four successive anion exchange columns: Source Q15, HiTrap DEAE FF and Mono Q 5/50 GL (GE Healthcare). Elution was performed with a 0–1-M NaCl gradient. Active fractions were combined, and buffer exchanged to 10 mM phosphate buffer (pH=7.4) containing 10 mM MgCl 2 using 10 kD Vivaspin 20 ml columns (GE Healthcare). Samples were then loaded onto a CHT ceramic hydroxyapatite column (Bio-Rad Laboratories Inc.); a linear gradient of 10–400 mM phosphate buffer was used for elution. The purified 20S proteasomes were analysed by SDS–PAGE, activity assays and MS analysis. Purification of 26S proteasomes Purification of the 26S was carried out using rat livers, which were homogenized in 300 ml buffer containing 50 mM Tris-HCL (pH 7.5), 250 mM sucrose, 10% glycerol, 2 mM DTT, 2 mM ATP, 1 mM EDTA and 5 U ml −1 Benzonase (Novagen). The extract was centrifuged at 1,000 g for 15 min. The supernatant was subjected to ultracentrifugation, initially at 145,000 g for 2.2 h and then at 150,000 g for 6 h. The pellet containing the 20S/26S proteasomes was resuspended in buffer containing 50 mM Tris-HCL (pH 7.5), 10% glycerol, 2 mM DTT, 2 mM ATP and 1 mM EDTA and loaded on Source-15Q anion exchange 55 ml column (GE Healthcare). The 20S and 26S proteasomes were separated by step elution of a 0–1-M NaCl gradient. Fractions containing the 26S proteasome were identified by SDS–PAGE, and by their ability to hydrolyse the fluorogenic peptide Suc-LLVY-AMC. The 26S proteasome-containing fractions were combined, and buffer exchanged to 10 mM phosphate buffer (pH 7.4) containing 10 mM MgCl 2 , using 10 kD Vivaspin 20 ml columns (GE Healthcare). Samples were then loaded onto a CHT ceramic hydroxyapatite column (Bio-Rad); a step gradient of 10–400 mM phosphate buffer was used for elution. The purified 26S proteasomes were analysed by SDS–PAGE and an in-gel activity assay using 4% native-PAGE. Native gels were run for 3.5 h at 120 V at 4 °C, using Tris-Glycine Running Buffer (25 mM Tris, 190 mM Glycine, pH 8.3) supplemented with 2 mM ATP and 2 mM DTT. The 26S proteasome samples were combined and concentrated, buffer exchanged to 100 mM phosphate buffer (pH 7.4) containing 10% glycerol, 5 mM MgCl 2 , 2 mM DTT and 2 mM ATP, using 10 kD Vivaspin 20 ml columns (GE Healthcare), and stored at −80 °C after snap-freezing in liquid nitrogen. Purification of recombinant DJ-1 WT and DJ-1 C106A The BL21(DE3) strain of E. coli was transformed with a pET-15b-hDJ-1 vector harbouring the full-length complementary DNAs of human DJ-1 WT or DJ-1 C106A . Cells were grown at 37 °C to an optical density of 0.45, at 600 nm, in 700 ml LB medium supplemented with 100 μg ml −1 ampicillin. Protein expression was induced by the addition of 0.4 mM isopropyl-β- D -thiogalactoside for 2.5 h. Cells were harvested by centrifugation for 20 min at 5000 g and resuspended in 50 ml of 50 mM Tris-HCl (pH 7.4), 2 mM EDTA, 1 mM DTT, 1 mM PMSF and a protease inhibitor cocktail (Complete, Roche). Cells were lysed in a French Press, centrifuged for 10 min at 5000 g and the lysate was passed through a Source-15Q anion exchange 55 ml column (GE Healthcare) pre-equilibrated with 50 mM Tris-HCl (pH 7.4) and 1 mM DTT. After lysate loading, proteins were eluted with 200 ml of 50 mM Tris-HCl (pH 7.4) and 1 mM DTT. Fractions (50 ml) were collected and DJ-1-containing fractions (eluted after 150–200 ml) were concentrated, using a 3-kDa Amicon Ultra column (Millipore). The concentrated DJ-1 sample was then loaded onto a gel filtration column (Superdex 200, 10/300 GL, GE Healthcare), pre-equilibrated with 50 mM Tris-HCl (pH 7.4), 300 mM NaCl and 1 mM DTT. DJ-1-containing fractions were combined, concentrated, frozen in liquid nitrogen and stored at −80 °C. Proteasome activity assay To monitor the relative activity levels of the 20S and 26S proteasomes during the purification steps, their proteolytic activity was assayed by measuring the hydrolysis of 100 μM of the proteasome fluorogenic substrate, Suc-LLVY-AMC (Boston Biochem), in the presence or absence of 0.02% SDS. In brief, between 10 and 20 pmols of samples containing the 20S or 26S proteasome were incubated in the dark in 100 μl Suc-LLVY-AMC solution, at 30 °C for 15–30 min. To stop the reaction, 200 μl SDS 1% was added to the mixture. After incubation, fluorescence of hydrolysed AMC groups was measured with a microplate reader (Infinite 200, Tecan Group), using an excitation filter of 380 nm and an emission filter of 460 nm. To determine whether DJ-1 influences the catalytic activity of the 20S proteasome, activity assays were performed in the presence and absence of DJ-1 or MG132. Purified 20S proteasomes (400 nM) were incubated overnight with or without 4.5 μM DJ-1 or 9 μM MG132. Subsequently, 4 μl of the mix was diluted into 50 μl activity buffer containing HEPES (25 mM; pH 7.4) and 200 μM Suc-LLVY-AMC, in the presence or absence of 0.02% SDS. Samples were incubated in the dark, at 30 °C for 15–30 min. To stop the reaction, 200 μl 1% SDS was added and fluorescence of hydrolysed AMC groups was measured, as described above. For the in-gel proteasome activity assay, 4% native-PAGE gels were soaked in 5 ml of 25 mM Tris-HCl (pH 7.4) supplemented with 100 μM Suc-LLVY-AMC. Gels were incubated in the dark at 30 °C for 15–30 min. After incubation, the gels were imaged under ultraviolet light. DJ-1 WT or DJ-1 C106A (300 pmol) was preincubated overnight with the 20S proteasome (15:1, DJ-1:20S molar ratio) at 4 °C. When indicated, MG132 was added to a final concentration of 9 μM. Degradation substrates (80 pmol α-synuclein, 560 pmol Cp53, 180 pmol NQO1 P187S , 184 pmol calmodulin and 184 pmol oxidized calmodulin) were then added. Reaction volumes were adjusted to 56 μl with HEPES buffer (50 mM; pH 7.4), and the mixture was incubated at 37 °C for 2 h. At different time points, 10 μl degradation reaction mix was removed and flash frozen in liquid nitrogen. The samples were boiled with 5 × x Laemmli sample buffer and loaded onto a 15% SDS–PAGE gel. Substrate levels were detected by Coomassie Blue Staining (for Cp53, α-synuclein and calmodulin) or immunoblot assays (NQO1 P187S and DJ-1). For the oxidation of DJ-1 WT and DJ-1 C106A , 6 nmol of the proteins were diluted in phosphate buffer (50 mM; pH 5.7) and incubated for 2 h at 37 °C with different concentrations of H 2 O 2 , as indicated. After oxidation, the proteins were dialysed three times against phosphate buffer (50 mM, pH 5.7). Oxidation of calmodulin (2 mg ml −1 , Sigma #P1431) was carried out by dissolving the protein in 0.1 M KCl, 50 mM HEPES, 1 mM MgCl 2 and 0.1 mM CaCl 2 , followed by the addition of 156 μl of H 2 O or 100 mM hydrogen peroxide. After 24 h incubation at 25 °C, the sample was dialysed twice in double-distilled water, titrated with ammonium bicarbonate to pH 7.7 and the protein concentration was determined. Quantitative image analysis of the degradation assays was carried out by measuring the band intensities with ImageJ software (NIH), and using the resulting values to determine the change in intensity with respect to T0, after reduction of background intensity. Each value represents an average of data from at least three experiments±s.d. Binding assays of DJ-1/proteasome DJ-1 WT (30 pmol) was preincubated overnight with 20S/26S proteasomes at a 1:1 molar ratio, in 50 μl of 50 mM HEPES buffer supplemented with 10% glycerol, 2 mM ATP and 2 mM DTT, at 4 °C. Samples were then loaded onto 4% native-PAGE gels and run for 3.5 h, 120 V at 4 °C, using Tris-glycine running buffer (25 mM Tris, 190 mM glycine, pH 8.3) supplemented with 2 mM ATP and 2 mM DTT. The DJ-1/20S/19S subunits were identified by western blot analysis using anti-α4, RPN2 and DJ-1 antibodies, as indicated above, and by an in-gel proteasome activity assay. MST of the interactions between DJ-1 and the 20S proteasome or Cp53, were measured on a Monolith NT.115 instrument (Nanotemper Technologies) [41] . DJ-1 WT and DJ-1 C106A were labelled with NT-647 fluorescent dye, using the Nanotemper Technologies labeling kit, according to the manufacturer’s instructions. Unlabelled 20S proteasome was serially diluted from 1–4 μM to 0.03–0.12 nM, while Cp53 was serially diluted from 18 μM to 1.1 nM. Measurements were performed in the presence of 50–75 nM of labelled DJ-1 WT or DJ-1 C106A , at room temperature, in phosphate buffer (0.2 M; pH 7.4), using 50%-70% LED power and 40% MST power. Data analysis was performed with Nanotemper analysis software. Each measurement was repeated three times. Cell lines and treatments HeLa cells were purchased from Cell Lines Service, Germany. The mouse fibroblast cell line A31N-ts20 BALB/c was obtained from Yosef Shaul (Weizmann Institute) and HEK293 cells, stably expressing the proteasome β4 subunit tagged with C-terminal FLAG were obtained from Chaim Kahana (Weizmann Institute). Cells were cultivated in Dulbecco’s Modified Eagle’s Medium supplemented with 10% fetal calf serum (FCS), penicillin–streptomycin, sodium-pyruvate, non-essential amino acids (Biological Industries) and MycoZap (Lonza) according to manufacturer’s instructions, in a humidified incubator at 32 °C (for A31N-ts20 BALB/c) or 37 °C (for HeLa and HEK293), in a 5% CO2 controlled atmosphere. HEK293 cells were supplemented with 1 mg ml −1 Puromycin. For silencing experiments, the following siRNAs were used: Dharmacon siGenome mouse PARK7 (M-050181-01-0005), Dharmacon siGenome non-targeting siRNA Pool #2 (D-001206-14-05) and Dharmacon siGenome Human PARK7 (M-005984-00-0005). JetPrime transfection reagent (Polyplus-transfection SA) was used for transfection of HeLa cells, according to the manufacturer’s instructions. After 24 h, the growth medium was replaced with medium containing reduced FCS (2%). A31N-ts20 BALB/c cells were transfected by electroporation using a NEPA21 electroporator (Nepa Gene Co., Ichikawa-City, Japan). For electrotransfection, 7.5 × 10 5 cells were mixed with 7.5 μg plasmid and/or 150 pmol of siRNA, and transfected according to the manufacturer’s instructions, using a poring pulse of 125 V for 5 ms. After electroporation, cells were cultured at 32 °C for 24 h; the growth medium was then replaced with medium containing reduced FCS (2%). Unless otherwise indicated, following 48 h of incubation at 32 °C, cells were transferred to 39 °C for another 24 h. Seventy-two hours post transfection, the cells were collected and lysed in modified RIPA buffer containing 50 mM HEPES (pH 7.6), 150 mM NaCl, 1% NP-40, 0.25% Na-deoxycholate, protease inhibitors (1 mM PMSF, 1 mM benzamidine, 1.4 μg ml −1 pepstatin A) and phosphatase inhibitors (1 mM Na-ortho-vanadate, 1 mM β-glycerophosphate and 2.5 mM Na-pyrophosphate). For western blot analysis, similar amounts of proteins were loaded (between 10 and 30 μg per sample). The gene-silencing effect of the siRNA treatment was calculated by dividing the band intensities of the treatments by those of the negative controls (NT siRNA or CFP), after reduction of background intensity. To evaluate the degradation rate of α-synuclein in cells depleted of DJ-1 at restrictive temperatures, A31N-ts20 BALB/c cells were transfected with siRNA against DJ-1 or non-targeting siRNA and cultured at 32 °C for 24 h; the growth medium was then replaced with medium containing reduced FCS (2%). Following 48 h of incubation at 32 °C, the cells were moved to 39 °C and incubated for another 24 h. Seventy-two hours post transfection, 200 μg ml −1 CHX were added for up to 100 min. Cells were collected at different time points and analysed by western blot, as indicated. Relative α-synuclein levels were calculated by dividing the band intensities at each time point by the intensity level at T0, after reduction of background intensity. Bars represent s.e.. All experiments were repeated between three and seven times. Oxidative stress was induced in A31N-ts20 cells transfected with siRNA against DJ-1 or non-targeting siRNA. Cells were then cultured at 32 °C for 48 h and then treated with 100 μM DEM. Subsequently, the cells were collected at different time points and analysed by western blot, as indicated. The change in protein levels was quantified by dividing the band intensities at 24 h after induction of oxidative stress, by the intensity level at T0 (defined as 100%), after reduction of background intensity. Values are an average of three independent experiments, errors represent s.e. Cell fractionation For cell fractionation, ~0.5 × 10 6 cells were resuspended in 0.2 ml hypotonic buffer A, containing 10 mM HEPES (pH 7.6), 10 mM KCl, 1.5 mM MgCl 2 , with phosphatase inhibitors, 0.5% NP-40 and protease inhibitors (0.26 mM PMSF, 1 mM benzamidine, 1.4 μg ml −1 pepstatin A) and incubated on ice for 10 min. Then, 5 μl of 10% NP-40 was added and cells were vortexed for 10 s. The cytosolic fraction was separated from the nuclei by centrifugation at 650 g for 3 min and further clarified by centrifugation at 10,000 g for 10 min. The nuclear pellet was washed in 0.1 ml buffer A and nuclei were pelleted at 450 g for 2 min. Nuclei were then resuspended in 0.1 ml hypertonic buffer CSK, containing 20 mM HEPES (pH 7.6), 100 mM NaCl, 300 mM sucrose, 3 mM MgCl 2 , 1 mM CaCl 2 , with or without phosphatase inhibitors, 0.5% Triton-X-100 and protease inhibitors and incubated on ice for 3 min. The nucleoplasmic fraction was separated by centrifugation at 5,000 g for 5 min. The pellet was resuspended in 0.08 ml hypertonic CSK buffer and incubated at room temperature for 15 min with 2,000 gel units of micrococcal nuclease (NEB). Chromatin-bound proteins were released from the DNA by addition of 0.02 ml of 1 M ammonium sulfate on ice, followed by centrifugation at 5,000 g for 5 min. Nucleoplasmic and chromatin-bound fractions were combined. Immunoprecipitation HEK293 cells stably expressing the FLAG-β4 subunit were plated in six 15-cm dishes, at a density of 1.5 × 10 6 cells per dish and grown for 24 h. Cells were collected by trypsinization, combined, washed in PBS and resuspended in 1 ml lysis buffer (20 mM Tris (pH 7.4), 10% glycerol, 10 mM NaCl, 3 mM MgCl 2 , 1 mM ATP) and protease inhibitors (1 mM PMSF, 1 mM benzamidine, 1.4 μg ml −1 pepstatin A). Cells were incubated on ice for 15 min and homogenized in a glass-Teflon homogenizer for 40 strokes. Lysate was cleared by centrifugation at 10,000 g for 10 min at 4 °C. For IP using anti-DJ-1 or antiRPN2 antibodies, 1 mg protein was diluted in 500 μl lysis buffer. NaCl concentration was adjusted to 150 mM. Proteins were precleared using 35 μl Protein G Sepharose (GE Healthcare), for 1 h at 4 °C, at a gentle rotation. The beads were discarded and the lysate was rotated overnight at 4 °C in the presence of 10 μl DJ-1 goat antibody or 5 μl anti-RPN2 antibody. The following morning, 35 μl Protein G Sepharose beads (GE Healthcare) were added, and lysate was rotated for 2 h at 4 °C. The beads were then washed three times in lysis buffer containing 150 mM NaCl and boiled in 100 μl protein sample buffer. For IP using anti-FLAG affinity gel, 1 mg protein was diluted in 500 μl lysis buffer. NaCl concentration was adjusted to 150 mM, and rotated overnight at 4 °C in the presence of 50 μl anti-FLAG M2 affinity gel (Sigma). The following morning, beads were washed three times with lysis buffer containing 150 mM NaCl and boiled in 100 μl protein sample buffer. Native mass spectrometry analysis Nanoflow electrospray ionization MS and tandem MS experiments were conducted under non-denaturing conditions on a QToF Q-Star Elite instrument (MDS Sciex, Canada), modified for improved transmission of large non-covalent complexes. Before MS analysis, 20 μl of up to 100 μM sample was buffer exchanged into 0.5–1 M ammonium acetate (pH 7.5), using Bio-Spin columns (Bio-Rad). Sample concentrations were determined by ultraviolet absorbance. Assays were performed in positive ion mode and conditions were optimized to enable the ionization and removal of adducts, without disrupting the non-covalent interactions of the proteins tested. In tandem MS experiments, the relevant m / z values were isolated and argon gas was admitted to the collision cell. Spectra are shown with minimal smoothing, and without background subtraction. Typically, aliquots of 1.5 μl of sample were electrosprayed from gold-coated borosilicate capillaries prepared in-house. The following experimental parameters were used: capillary voltage up to 1.1 kV, declustering potential up to 220 V, focusing potential up to 240 V, a second declustering potential of 15 V, collision energy of between 20 and 200 V and an MCP of 2,350 V. How to cite this article: Moscovitz, O. et al. The Parkinson’s-associated protein DJ-1 regulates the 20S proteasome. Nat. Commun. 6:6609 doi: 10.1038/ncomms7609 (2015).